Abiotic methanogenesis from organosulphur compounds under ambient conditions Methane in the environment is produced by both biotic and abiotic processes. Biomethanation involves the formation of methane by microbes that live in oxygen-free environments. Abiotic methane formation proceeds under conditions at elevated temperature and/or pressure. Here we present a chemical reaction that readily forms methane from organosulphur compounds under highly oxidative conditions at ambient atmospheric pressure and temperature. When using iron(II/III), hydrogen peroxide and ascorbic acid as reagents, S-methyl groups of organosulphur compounds are efficiently converted into methane. In a first step, methyl sulphides are oxidized to the corresponding sulphoxides. In the next step, demethylation of the sulphoxide via homolytic bond cleavage leads to methyl radical formation and finally to methane in high yields. Because sulphoxidation of methyl sulphides is ubiquitous in the environment, this novel chemical route might mimic methane formation in living aerobic organisms. The greenhouse gas methane (CH 4 ) is the most abundant reduced organic trace gas in the atmosphere and has an important role in tropospheric and stratospheric chemistry. Various sources of CH 4 are known to exist in nature, and, recently, the number of suggested biological sources has been increased [1] , [2] , [3] , [4] . However, the mechanism of CH 4 formation in eukaryotes still needs to be elucidated and precursor compounds to be identified. In general, natural formation of CH 4 —so-called methanogenesis—can be classified into biotic and abiotic types. Biotic methanogenesis is usually associated with archaea, living under anaerobic conditions in wetlands, rice fields, landfills or the gastrointestinal tracts of ruminants and termites. Abiotic formation of CH 4 has been reported to occur under conditions that require high pressure and/or temperature, for instance, during biomass burning or serpentinization of olivine, under hydrothermal conditions in the oceans’ depths or below tectonic plates [5] , [6] , [7] . In the chemical industry, CH 4 is often produced from carbon monoxide and hydrogen gas under elevated pressure and temperature ( cf . Fischer–Tropsch synthesis). Over the past few years, CH 4 formation without the help of methanogens has also been observed in living biological systems such as plants [1] , [8] , [9] , [10] , fungi [2] and animals [3] , [4] . Whereas the biochemistry of methanogenesis in microbes (procaryotes) is well described [11] , [12] , possible pathways of aerobic CH 4 generation from plants, fungi and animals (eukaryotes) have yet to be determined. A comprehensive understanding of all environmentally important CH 4 sources and sinks, as well as the parameters that control emissions is a prerequisite to fully understanding the global biogeochemical cycle of CH 4 . In particular, CH 4 formation and emissions by both dead and living plants [8] has been intensely discussed in recent years [1] , [13] , [14] . It has been shown that CH 4 can be produced abiotically from plant material by exposing it to ultraviolet (UV) irradiation [15] , [16] , [17] , [18] . A reaction of reactive oxygen species (ROS) with methoxyl groups of pectic polysaccharides was suggested as a possible route to CH 4 formation under UV radiation [19] . On the other hand, several recent studies [2] , [9] , [10] , using 13 C-labelled plant and fungal species, have demonstrated that there is also continuous formation of CH 4 in living plants and fungi without any microbial contribution. It has been hypothesized that hetero-bonded methyl groups of biomolecules such as the sulphur-containing amino acid methionine or the ammonium salt choline might be carbon precursors of CH 4 in living cells [1] , [2] , [3] , [10] , [20] , [21] , [22] . Althoff et al. [23] recently showed that ascorbic acid (ASC) produces small amounts of CH 4 when using a combination of an iron oxyhydroxide and hydrogen peroxide (H 2 O 2 ) as an oxidizing system. Biomimetic iron complexes are generally designed to mimic the biocatalytic activity of mono- and di-oxygenase enzymes [24] . This includes the oxidative metabolism of sulphides to yield sulphoxides, sulphones and S-dealkylation products (thiols and aldehydes). However, no chemical pathway producing CH 4 under these conditions has been described so far. In this work, we investigate a chemical reaction system containing iron(II/III), H 2 O 2 and ASC that uses organic compounds with hetero-bonded methyl groups for the generation of CH 4 under ambient (1,000 mbar and 22 °C) and aerobic (~\n21% O 2 ) conditions. In particular, several S-methyl substituted sulphides, sulphoxides and sulphonium salts such as L -methionine (MET), S-adenosylmethionine (SAM), dimethylsulphoniopropionate (DMSP) and dimethyl sulphoxide (DMSO) are studied. Compounds with nitrogen and oxygen hetero-bonded methyl groups such as choline chloride (CC) and guaiacol (GU; 2-methoxyphenol) are also investigated. Most of the selected compounds are known to have a key role in bio-methylation reactions and methyl group metabolism of plants, fungi and animals [25] ( Supplementary Note 1 ). We describe a chemical reaction that readily forms CH 4 from organosulphur compounds under highly oxidative conditions. We hypothesize that this novel chemical route might mimic CH 4 formation in living aerobic organisms such as plants, fungi, algae and mammals. Formation of CH 4 from organosulphur compounds A selection of organic compounds with hetero-bonded methyl groups were investigated to serve as possible CH 4 precursors when ASC, ferrihydrite (FH; 5Fe 2 O 3 ·9H 2 O) and H 2 O 2 were used as reagents in aqueous solution under ambient conditions. 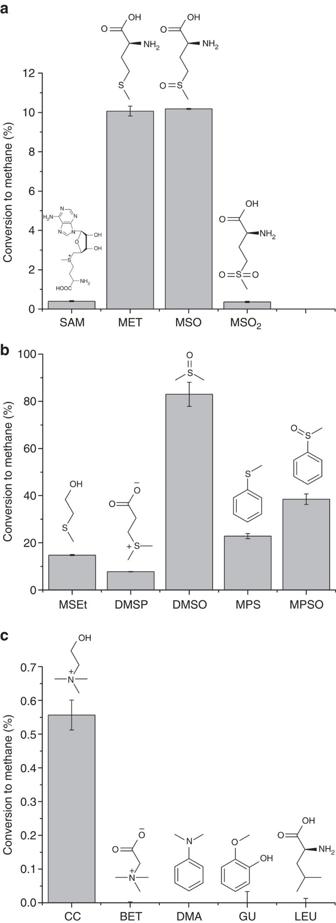Figure 1: CH4formation from different methyl substituted substrates. Among methylated substrates used are (a) S-adenosylmethionine (SAM),L-methionine (MET), methionine sulphoxide (MSO) and methionine sulphone (MSO2); (b) 2-(methylthio)ethanol (MSEt), dimethylsulphoniopropionate (DMSP), dimethyl sulphoxide (DMSO), methyl phenyl sulphide (MPS) and methyl phenyl sulphoxide (MPSO); and (c) choline chloride (CC), betaine (BET),N,N-dimethylaniline (DMA), guaiacol (GU) and leucine (LEU). Values show molar conversion of methyl substituted substrates as percentages. The initial amounts of reactants were 50 μmol ASC, 4 μmol FH, 100 μmol H2O2and 0.5 μmol methylated substrates (0.025 μmol DMSO) in 1 ml total volume (H2O), and headspace 360 ml, ambient temperature and ambient atmosphere. Data show mean value±s.d. (n=3); reaction time of 30 h. The pH in the medium was in the range of 2.9–3.1. Figure 1 shows the conversion/yield of CH 4 formed from each of the investigated compounds. All substrates with sulphur-bonded methyl groups showed significant CH 4 production but with tremendously varying yields, ranging from 0.4 to 83% ( Fig. 1a,b ) under the applied conditions. MET and its sulphoxidation product, methionine sulphoxide (MSO), showed similar yields of ~\n10%, whereas methionine sulphone (MSO 2 ), the further oxidized form of MSO, showed little evidence of CH 4 formation (<0.4%). SAM, a sulphonium derivative of MET, also showed little conversion to CH 4 (~\n0.4%). A high yield of CH 4 (~\n40%) was observed for the aromatic compound methyl phenyl sulphoxide (MPSO). Methyl phenyl sulphide (thioanisole) showed a somewhat lower yield of CH 4 (~\n23%). DMSP and 2-(methylthio)ethanol produced CH 4 at conversion rates (8% and 15%, respectively) that were in a similar range to those observed for MET and MSO. DMSO produced the highest CH 4 conversion rate of 83%. CH 4 formation was not observed in any experiment in the absence of H 2 O 2 or iron minerals or ASC. Figure 1: CH 4 formation from different methyl substituted substrates. Among methylated substrates used are ( a ) S-adenosylmethionine (SAM), L -methionine (MET), methionine sulphoxide (MSO) and methionine sulphone (MSO 2 ); ( b ) 2-(methylthio)ethanol (MSEt), dimethylsulphoniopropionate (DMSP), dimethyl sulphoxide (DMSO), methyl phenyl sulphide (MPS) and methyl phenyl sulphoxide (MPSO); and ( c ) choline chloride (CC), betaine (BET), N , N -dimethylaniline (DMA), guaiacol (GU) and leucine (LEU). Values show molar conversion of methyl substituted substrates as percentages. The initial amounts of reactants were 50 μmol ASC, 4 μmol FH, 100 μmol H 2 O 2 and 0.5 μmol methylated substrates (0.025 μmol DMSO) in 1 ml total volume (H 2 O), and headspace 360 ml, ambient temperature and ambient atmosphere. Data show mean value±s.d. ( n =3); reaction time of 30 h. The pH in the medium was in the range of 2.9–3.1. Full size image CH 4 formation from DMSO has been described before [26] , [27] , [28] : hydroxyl radicals, produced via radiolysis of water or via Fenton’s reaction, have been shown to react with DMSO to produce methyl radicals. This reaction leads to CH 4 , ethane (C 2 H 6 ), methanol and/or formaldehyde, depending on the reaction conditions [26] , [27] , [28] , [29] . However, under conditions used in our experiments (iron(II/III), ASC and H 2 O 2 ), when FH is replaced by water-soluble iron salts that are believed to produce hydroxyl radicals (Fenton’s reaction), very little CH 4 production was observed (<1%; Supplementary Fig. 1 ). This observation is consistent with a reaction pathway for CH 4 formation from DMSO that differs from that described previously. Specifically, it appears that there must be another oxidant since hydroxyl radicals are known to be quenched by the antioxidant ASC [30] . Compounds with N -methyl and O -methyl groups such as betaine, N , N -dimethylaniline, and GU showed no measurable formation of CH 4 in our experiments ( Fig. 1c ). The only exception was CC, a quaternary ammonium salt, that showed little CH 4 conversion (≈0.6%). No CH 4 formation was found when using the amino acid leucine. To unravel the reaction pathway of CH 4 formation, we focused on MET and MSO since they both showed considerable CH 4 formation at similar yields, and also have a vital role in most living organisms. Identification of the CH 4 precursor carbon atom We expected the S-methyl group of MET to be the carbon precursor of CH 4 . This was tested with positionally labelled 13 CH 3 -MET and measuring stable carbon isotope values ( δ 13 C values) of CH 4 , using gas chromatography combustion isotope ratio mass spectrometry (GC-C-IRMS). When 13 CH 3 -MET (~\n2% 13 C) was used for the reaction, the δ 13 C values of CH 4 changed drastically to more positive values (from −47 to +763‰ versus Vienna Pee Dee Belemnite, VPDB), and reflected the anticipated δ 13 C values when considering the isotopically labelled methyl group as the CH 4 precursor. These results unambiguously identify the sulphur-bonded CH 3 group of methionine as the carbon precursor of CH 4 . Parameters that control CH 4 production The amount of CH 4 produced was found to vary according to the type of iron species, concentrations of H 2 O 2 and ASC, pH and gas atmosphere used. In addition to FH (5Fe 2 O 3 ·9H 2 O), we investigated other oxyhydroxides such as goethite, α-FeO(OH), lepidocrocite, γ-FeO(OH), the iron oxide haematite (HT; Fe 2 O 3 ) and soluble Fe 2+ and Fe 3+ salts ( Fig. 2 and Supplementary Table 1 ). All iron species investigated showed significant CH 4 formation in the reaction with MET, ASC and H 2 O 2 , but there were large differences in conversion efficiency between the iron minerals and the soluble Fe 2+ and Fe 3+ salts. After a reaction time of 5 h, FH showed the highest CH 4 formation of ~\n5%, followed by the other iron minerals (~\n3%), whereas formation of CH 4 induced by the Fe 2+ and Fe 3+ salts was much lower (~\n0.5%). The yields of CH 4 increased further to values ranging from 11 to 15% for the iron minerals, with HT showing the highest formation, whereas the Fe 2+ and Fe 3+ salts showed a considerably lower conversion ratio of ~\n2–3%. After 48 h, for all iron species, no further CH 4 increase was observed. Since the core of the iron storage protein of many living systems, ferritin, has a structure similar to that of FH [31] , the iron oxyhydroxide FH was used for all further experiments. From Fig. 2 , it appears that the formation of CH 4 may depend on the kinetics of the dissolution process of the iron minerals, that is, on a low steady-state concentration of Fe 2+ in solution. However, a heterogenous process, involving the solid catalysts, might be also conceivable. 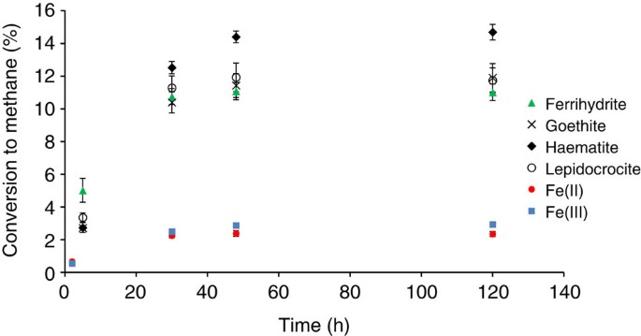Figure 2: Formation of CH4fromL-methionine (MET) using different iron species. The initial amounts of reactants were 50 μmol ASC, 40 μmol Fe (different species), 100 μmol H2O2and 0.5 μmol MET in H2O (1 ml total volume), and headspace 360 ml, ambient temperature and ambient atmosphere. Values measured after 30 h. Data show mean value±s.d. (n=3). The pH in the medium was in the range of 2.9–3.1. Figure 2: Formation of CH 4 from L- methionine (MET) using different iron species. The initial amounts of reactants were 50 μmol ASC, 40 μmol Fe (different species), 100 μmol H 2 O 2 and 0.5 μmol MET in H 2 O (1 ml total volume), and headspace 360 ml, ambient temperature and ambient atmosphere. Values measured after 30 h. Data show mean value±s.d. ( n =3). The pH in the medium was in the range of 2.9–3.1. Full size image A set of experiments was designed to maximize CH 4 production by altering the molar ratio of ASC and H 2 O 2 while maintaining a constant amount of FH and MET ( Supplementary Fig. 2 ). Maximum CH 4 formation was observed with a molar ratio of H 2 O 2 : ASC of 2:1 (50 μmol ASC and 100 μmol H 2 O 2 ). When adding MET to this ratio of ASC and H 2 O 2 , a linear correlation between CH 4 formation and the amount of added MET was observed ( Fig. 3 ). 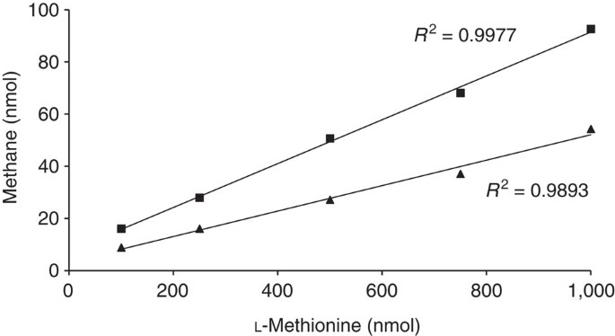Figure 3: Linear relationship between CH4formation and the amount of added methionine. Triangles and squares show CH4production after 5 and 30 h, respectively. The initial amounts of reactants were 50 μmol ASC, 4 μmol FH and 100 μmol H2O2, and varying amounts of MET in H2O with a total volume of 1 ml, headspace 360 ml, ambient temperature and ambient atmosphere. Data show mean value s.d. (n=6). Error bars lie within symbols. The pH in the medium was in the range of 2.9–3.1. Figure 3: Linear relationship between CH 4 formation and the amount of added methionine. Triangles and squares show CH 4 production after 5 and 30 h, respectively. The initial amounts of reactants were 50 μmol ASC, 4 μmol FH and 100 μmol H 2 O 2 , and varying amounts of MET in H 2 O with a total volume of 1 ml, headspace 360 ml, ambient temperature and ambient atmosphere. Data show mean value s.d. ( n =6). Error bars lie within symbols. The pH in the medium was in the range of 2.9–3.1. Full size image The influence of pH on CH 4 production was monitored in the pH range of 1–9. The highest yield of CH 4 was found at pH 3, the pH generally observed in our experiments ( Supplementary Fig. 3 and Supplementary Table 2 ). The influence of O 2 concentration (in the surrounding headspace) on the yield of CH 4 was also studied. Interestingly, production of CH 4 under ambient and anaerobic conditions was basically identical, whereas under a pure O 2 atmosphere the yield was reduced by ~\n50 % ( Supplementary Fig. 4 ). We measured the O 2 content of the headspace and aqueous solution in our standard reaction mixture (4 μmol FH, 50 μmol ASC, 100 μmol H 2 O 2 , 0.5 μmol MET, 1 ml H 2 O, headspace 360 ml containing ~\n21% O 2 , ambient temperature and ambient atmosphere) vessel over the entire reaction period of 30 h. Although the O 2 concentration in the headspace remained relatively constant (100% atmospheric air saturation) throughout the measurement period, the aqueous solution was found to be close to zero and then to rise gradually (ranging from 0 to 60% atmospheric air saturation; Supplementary Fig. 5 ). The low levels of O 2 found in aqueous solution can be explained by its rapid consumption by methyl radicals, which is discussed in much more detail below. 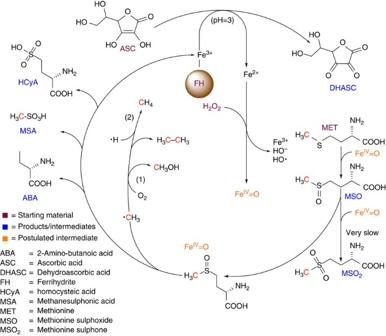Figure 4: Route of abiotic CH4formation. The ferryl species ([FeIV=O]2+, coloured in orange) is postulated to be primarily responsible for CH4formation (see text). The carbon atom from which CH4emerges is highlighted in light red. Starting materials are coloured in dark red (stoichiometric factors omitted). Postulated route of CH 4 formation Figure 4 shows a novel reaction mechanism for CH 4 formation from MET, which is in agreement with and supported by our experimental data. The central observations are as follows: (i) MET is oxidized to MSO, which then produces CH 4 and other products in the following reaction steps; and (ii) CH 4 originates from the methyl group of MET ( 13 C isotope labels are highlighted in red). Figure 4: Route of abiotic CH 4 formation. The ferryl species ([Fe IV =O] 2+ , coloured in orange) is postulated to be primarily responsible for CH 4 formation (see text). The carbon atom from which CH 4 emerges is highlighted in light red. Starting materials are coloured in dark red (stoichiometric factors omitted). Full size image In solution, ASC is deprotonated (p K a =4.37), leading in general to a pH value of ~\n3 in the solutions used for our experiments. Under these conditions, the crystalline FH is reductively dissolved by ASC, releasing slowly Fe 2+ to produce a low steady-state concentration of Fe 2+ over several hours. The Fe 2+ ions are oxidized by H 2 O 2 to produce Fe 3+ , [Fe IV =O] 2+ (ferryl species) and ·OH. The ·OH radicals might lead to unspecific radical reactions but they are trapped by ASC, which is transformed to dehydroascorbic acid. Experimentally, this is supported by the fact that little formation of CH 4 was observed from MET and DMSO when Fe 2+ or Fe 3+ salts were used as the iron source instead of FH ( Fig. 2 and Supplementary Fig. 1 ); under these Fenton-type conditions, the reaction should be fast and complete within a few minutes. Therefore, the low steady-state concentration of Fe 2+ (reductive dissolution of FH, formation of dehydroascorbic acid + 2H + + 2e − ) is of importance. An alternative oxidant in aqueous Fe 2+ /H 2 O 2 systems is [Fe IV =O] 2+ , and this ferryl species is known from nonhaeme iron enzymes and corresponding biomimetic oxidation catalysis [24] , [32] to be a powerful oxidant in aqueous solution [33] , [34] , [35] , [36] . Bispidine-type ligands have been shown to efficiently support the ferryl centre for oxidation catalysis. Thorough mechanistic studies of these systems have been reported (for structures of the ligands and ferryl complexes and more details of the model chemistry, see Supplementary Figs 6 and 7 , and Supplementary Notes 2 and 3 ) [37] , [38] . To support the proposed mechanistic scenario in Fig. 4 , we have therefore replaced FH in our test reaction (FH, H 2 O 2 , ASC and MET) by an iron bispidine complex ([(L 1 )Fe IV =O] 2+ ) and shown that analogous products and product ratios are produced under otherwise identical experimental conditions ( Supplementary Table 3 ). Based on known iron bispidine chemistry, this indicates that a ferryl ion transfers the oxo group to MET forming MSO [39] , and a second ferryl species may react as electrophile with the methyl group of MSO to produce a ·CH 3 radical, similar to known reactivities of the ferryl species with C–H bonds [40] . Importantly, the sulphoxidation of a thioether (for example, MET or thioanisole) is much faster than that of the sulphoxide product MSO (or MPSO) to form the corresponding sulphone (MSO 2 or methyl phenyl sulphone; see Supplementary Figs 7 and 8 for a kinetic analysis of the thioanisole/MPSO example: the oxidation of the thioether is more than two orders of magnitude faster than that of the sulphoxide; methyl phenyl sulphone was found as a product but not quantified, that is, the oxidation of MPSO may lead to different products, for example, methyl phenyl sulphone (oxygen transfer), ·CH 3 radicals (CH 3 abstraction) or sulphoxide radical cations (electron transfer)). To further support this assumption, the produced ·CH 3 radicals were trapped with DMPO (5,5-dimethyl-pyrroline- N -oxide) and unambiguously characterized by electron paramagnetic resonance (EPR) spectroscopy (for details, see Supplementary Fig. 9 and Supplementary Note 4 ). Because of the high reactivity of the spin trap DMPO with radicals, all aqueous solutions, especially the DMPO solution, were carefully degassed. However, because of disproportionation and radical reactions, aqueous H 2 O 2 solutions contain some O 2 and ·OH radicals ( Supplementary Fig. Note 4 ). Therefore, in aqueous solutions of the spin trap (DMPO, 100 mmol), H 2 O 2 (0.25 mmol), MPSO (2.5 mmol) and iron(II)triflate (0.25 mmol) both ·OH and ·CH 3 radicals are detected, the latter only as a minor species ( Fig. 5a ). When ASC (0.25 mmol) was added, the EPR spectrum shows the ·CH 3 radicals as the major species since ASC traps ·OH radicals more efficiently than ·CH 3 radicals ( Fig. 5b ). This supports our interpretation that the formation of CH 4 is induced by ferryl species rather than ·OH radicals, since these are efficiently quenched under the conditions of our experiments. 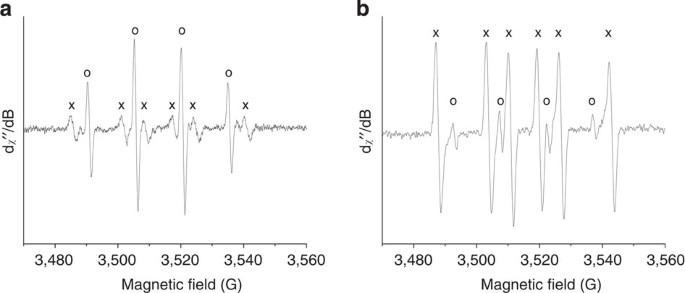Figure 5: X-band EPR spectra of DMPO-OH and DMPO-CH3. X-band EPR spectrum of (a) DMPO-OH (o;giso=2.00585,aN=aH=14.91 G,ν= 9.863566 GHz) and (b) DMPO-CH3(x;giso=2.00574,aN=16.06 G,aH=23.05 G,ν= 9.869031 GHz) in H2O at 298 K (seeSupplementary Informationfor more experimental and computer-simulated spectra and experimental details). Figure 5: X-band EPR spectra of DMPO-OH and DMPO-CH 3 . X-band EPR spectrum of ( a ) DMPO-OH (o; g iso =2.00585, a N = a H =14.91 G, ν = 9.863566 GHz) and ( b ) DMPO-CH 3 (x; g iso =2.00574, a N =16.06 G, a H =23.05 G, ν = 9.869031 GHz) in H 2 O at 298 K (see Supplementary Information for more experimental and computer-simulated spectra and experimental details). Full size image The formation of methyl radicals is further supported by the formation of C 2 H 6 ( 13 C-labelled). However, C 2 H 6 is, as expected, formed in very low quantities, with a C 2 H 6 /CH 4 ratio below 0.01. It has been shown that formation of C 2 H 6 by the recombination of methyl radicals occurs in water and depends on the experimental parameters [27] , [41] , [42] . In those studies, much higher C 2 H 6 /CH 4 ratios (>0.1) were reported because of the fast kinetics (for example, ·OH radical formation by water radiolysis), generating a higher steady-state concentration of methyl radicals. The slow formation of Fe 2+ from FH and of [Fe IV =O] 2+ by oxidation with H 2 O 2 leads to a small steady-state concentration of ·CH 3 radicals that might explain the almost exclusive CH 4 formation (low C 2 H 6 /CH 4 ratio) observed in our study: a fast oxidation of Fe II with H 2 O 2 leads to much lower CH 4 formation in the investigated system, as was shown by the experiments using Fe 2+ and Fe 3+ salts and MET and DMSO as thioethers ( Fig. 2 and Supplementary Fig. 1 ). The observation that the bispidine–ferryl complexes yield similar products and product ratios under similar conditions indicates that the observed reaction with FH is a homogenous process. There are competing oxidation reactions of the methyl radical with H 2 O 2 or O 2 , yielding methanol, formaldehyde and formic acid [41] , [42] . Specifically, the reaction of ·CH 3 radicals with O 2 is very likely [43] . Formation of methanol was confirmed during our reaction but not quantified so far. The reaction of ·CH 3 radicals with O 2 , forming methanol and other oxidative products (for example, peroxides and formaldehyde) [42] , [43] , is ~\n3–5 orders of magnitude faster than that with other substrates present, leading to CH 4 (H atom transfer from alkanes, alkyl groups, ASC and H 2 O 2 ), that is, CH 4 is only produced at low concentration of O 2 (dioxygen shunt, pathways (1) and (2) in Fig. 4 ; for kinetic parameters, see Notre Dame Radiation Laboratory (NDRL)/National Institute of Standards and Technology (NIST) solution kinetics database, http://kinetics.nist.gov/solution/ ). This is supported by the low yield of CH 4 in a pure dioxygen atmosphere ( Supplementary Fig. 4 ) and also explains the observed maximum yield of 20% CH 4 relative to MET. Importantly, our mechanism indicates that CH 4 formation is possible under ambient atmosphere but does not require O 2 , which agrees with the observation that our standard reaction also produces CH 4 under N 2 (similar yield; Supplementary Fig. 4 ). We suggest that the reaction is induced by ferryl species rather than ·OH radicals. This emerges from the fact that ASC efficiently quenches the ·OH radicals, and that the model reaction with the bispidine–ferryl complexes, which are mechanistically well studied, produce under similar conditions similar amounts of the respective products, specifically of CH 4 . Further products identified by their accurate mass using liquid chromatography–time of flight MS (LC–TOFMS) during the reaction ( Supplementary Note 5 ) are also shown in Fig. 4 . Obviously, both S–C bonds of MSO may be attacked by the ferryl group. Thus, formation of CH 4 and 2-amino-butanoic acid were assumed to result from a reduction of the carbon atoms, whereas methanesulphonic acid identified by high-performance liquid chromatography (HPLC) and homocysteic acid were oxidation products. Two additional products having accurate mass values and adducts consistent with empirical formulae C 4 H 9 NO 3 S and C 4 H 8 O 4 S were identified by LC–TOFMS. Although these formulae are compatible with structures such as the previously unreported homocysteine sulphenic acid and 2-hydroxy-4-sulphenobutanoic acid; sulphenic acids are normally found to be highly reactive transient compounds that are difficult to detect and isolate unless stabilized by steric hindrance [44] or intramolecular H-bonding involving a seven-membered ring [45] . However, in view of the known instability of most sulphenic acids [44] , much stronger evidence will be required before the structures for the minor products can be confirmed and thus they are not shown as decay products in Fig. 4 . The detailed mechanism of the electrophilic attack of the ferryl species at the CH 3 –(S=O)–R bond(s), the kinetics of the two proposed pathways (formation of CH 4 , CH 3 OH and /or other products in our closed system and, in general, as a function of the reaction conditions), as well as a possible involvement of ·OH radicals clearly need detailed further studies, and these will involve density functional theory (DFT)-based computational and further experimental investigations. The results reported here show that CH 4 is formed from both dialkyl and alkyl aryl thioethers under highly oxidative conditions at ambient atmospheric pressure and temperature. High CH 4 yields were observed from both aliphatic and aromatic methyl sulphides and the corresponding sulphoxides. The applied iron species together with H 2 O 2 are known to catalyse a range of non-selective hydrocarbon oxidations. However, they also act as biomimetic ferryl systems to catalyse hydrocarbon oxidations with high chemo-, regio- and stereo-selectivity [24] , [46] . Ferryl species also catalyse heteroatom oxidation of methyl sulphides to yield sulphoxides and sulphones and S-dealkylation to give thiols and formaldehyde. Our experiments show that these systems can also support reductive demethylation of sulphoxides yielding CH 4 as the final dealkylation product at low local oxygen concentration. Methyl sulphides are present in the environment as both natural and anthropogenic products and metabolites from S -methyltransferase-catalysed methylation of thiols and their 1,2-disulphide precursors. The interaction of ASC with FH in particular has a strong biochemical connection, since the inorganic core of ferritin, nature’s Fe sequestration protein common to living organisms, is presumably FH. Ferritins are important iron storage and detoxification proteins that are widely distributed in living kingdoms. ROS, including H 2 O 2 , are continuously produced at different rates in biological systems due to biotic and abiotic stress reactions. Hence, our observations of the interaction of ASC with H 2 O 2 , FH and methyl sulphides and sulphoxides might have relevance to understanding CH 4 formation under oxidative conditions in biochemical systems such as in terrestrial and aquatic plants, fungi and mammals [1] , [2] , [3] , [4] , [10] . The sulphur-containing amino acid MET and the sulphonium salt DMSP are of particular global and biochemical importance. Methionine is known to be a key factor in many biochemical reactions in plants, fungi and animals, and it has been recently shown [2] to be a CH 4 precursor in fungi. However, so far methionine has not been shown to be a precursor of CH 4 in living plants. To test this hypothesis tobacco plants ( Nicotiana tabacum ) that were grown under sterile conditions were supplemented with positionally labelled MET, where only the methyl group (–S–CH 3 ) was enriched with 13 C atoms (99% 13 CH 3 ). For these isotope tracer experiments, leaves and roots of the tobacco plants were separately treated with 13 C-MET ( Fig. 6 ) at different concentrations. As expected, at time zero after initial treatment with labelled or unlabelled MET, all samples showed CH 4 stable carbon isotope values ( δ 13 C(CH 4 ) values) of approximately −46‰ (ranging from −45.4 to −47.1‰), closely reflecting the atmospheric background δ 13 C(CH 4 ) values of the laboratory air (−46.1±0.5‰). As also expected, δ 13 C(CH 4 ) values of the headspace of the tobacco plants containing unlabelled MET did not change significantly over the incubation period. In contrast, δ 13 C(CH 4 ) values in the headspace of the tobacco plants supplemented with 13 C-MET at different concentrations, both to the leaves and roots, showed a continuous increase over the entire incubation period clearly showing that the thio-methyl group acts as precursor of plant-derived CH 4 (for more details, see Supplementary Note 6 ). Although these experiments do not give information about the pathway of CH 4 formation in plants, they provide evidence that the thio-methyl group of MET is a precursor of CH 4 . 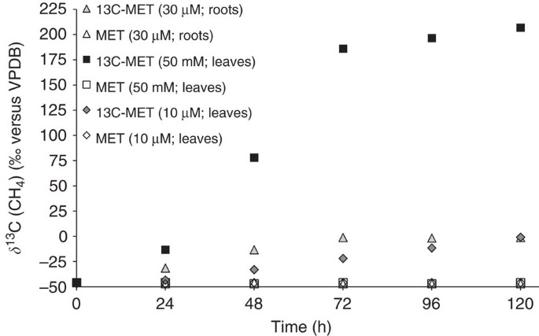Figure 6:δ13C values of CH4produced by tobacco plants supplemented with13C-MET. Black squares, diamonds and triangles show values measured for plants when treated with 50 mM (leaves), 10 μM (leaves) and 30 μM (roots)13C-labelled MET, respectively; white symbols are for the corresponding treatments with unlabelled MET. Figure 6: δ 13 C values of CH 4 produced by tobacco plants supplemented with 13 C-MET. Black squares, diamonds and triangles show values measured for plants when treated with 50 mM (leaves), 10 μM (leaves) and 30 μM (roots) 13 C-labelled MET, respectively; white symbols are for the corresponding treatments with unlabelled MET. Full size image Methionine residues in proteins are particularly sensitive to oxidation by ROS and thus have been suggested to defend against oxidative stress [47] . The sulphur-containing amino acids methionine and cysteine are more easily oxidized than the other amino acids. The oxidation of MET to MSO by H 2 O 2 is common in cells [48] , [49] . Peroxides, including H 2 O 2 , hydroperoxides and peroxy acids, are efficient oxidants of organic sulphides in aqueous solutions. For example, the oxidation of methionine groups by hydroperoxides is a major pathway for the degradation of therapeutic proteins. DMSP, an algal osmolyte that is abundant in marine phytoplankton and comprises 1–10% of the carbon in some algal species [50] , serves also as a precursor for the volatile compounds dimethyl sulphide (DMS) and DMSO in seawater. Thus, it could be envisaged that these thioethers and sulphoxides might be a direct precursor of CH 4 formed in oxic and suboxic waters, and could help to overcome the so-called ‘oceanic methane paradox’. The highest CH 4 formation rates might be expected from aerobic organisms particularly when under hypoxia. This important consideration is in agreement with previous results that showed enhanced CH 4 formation in animal cells under reduced oxygen content [3] , [4] . Finally, we suggest that the CH 4 pathway described herein might be considered as an ‘oxidative counterpart’ of the final step of biological CH 4 formation in methanogenic archaea where the methyl coenzyme M reductase catalyses the reaction between thioether methyl coenzyme M and the thiol N -(7-mercaptoheptanoyl)threonine 3- O -phosphate to give CH 4 and the mixed disulphide [51] . Compounds tested as methane precursor SAM, MET, MSO, MSO 2 , 2-(methylthio)ethanol, DMSP, DMSO, methyl phenyl sulphide, MPSO, CC, betaine, N , N -dimethylaniline, GU and leucine (LEU) were all tested for their potential to release CH 4 . An amount of 4 μmol FH (40 μmol Fe) was weighted into 1.5 ml crimp vials. These vials were then placed into the 360 ml vials that were sealed using a hole-type screw cap (Supelco, cat. no. 27187) fitted with a polytetrafluorethylen (PTFE)/silicone septum (Supelco, cat. no. 27188-U) before 0.5 μmol of the organic compound dissolved in 0.4 ml H 2 O, 50 μmol ASC dissolved in 0.5 ml H 2 O and 100 μmol H 2 O 2 in 0.1 ml H 2 O, were injected to each 1.5 ml vial through the septum. All samples were prepared under normal laboratory conditions. The samples were incubated at 22±2 °C for a time period of up to 120 h before CH 4 headspace analysis. Reagents Organic compounds and iron salts were obtained from Sigma, Deisenhofen, Germany, in the highest purity available. The iron minerals FH, goethite, HT and lepidocrocite were synthesized as prescribed by Schwertmann and Cornell [52] . Surface areas and particle sizes of the iron minerals are presented in the Supplementary Table 1 . Double distilled H 2 O filtered with an ELGA UHQ-II-MK3 was used for these investigations. CH 4 measurements Headspace (5 ml) from the sealed glass vials was sampled using a Hamilton gas syringe needle and analysed by a gas chromatograph (GC; column: 2 m, Ø =3.175 mm (inner diameter) high-grade steel tube packed with Molecular Sieve 5A 60/80 mesh from Supelco) equipped with a GC–flame ionization detector (Shimadzu GC-14B). Quantification of CH 4 was performed by direct comparison of peak area with that obtained with two reference standards containing 8.905 and 1.835 p.p.m. All samples were prepared in triplicate ( n =3) unless otherwise stated in the manuscript. Control samples (blanks) were prepared in a similar manner to that described for the samples but without the addition of methyl substituted substrates. The control measurements usually reflected the CH 4 background concentration of the laboratory (range 2–2.2 p.p.m.). Stable carbon isotope measurements δ 13 C values of CH 4 were measured by a GC-C-IRMS procedure. The GC-C-IRMS system consisted of a cryogenic pre-concentration unit directly coupled to an HP 6890N GC (Agilent Technologies, Santa Clara, USA), which is connected to a Delta PLUS XL isotope ratio mass spectrometer (ThermoQuest Finnigan, Bremen, Germany) via an oxidation reactor (ceramic tube (Al 2 O 3 ), length 320 mm, 0.5 mm i.d., with oxygen activated Cu/Ni/Pt wires inside, reactor temperature 960 °C) and a GC Combustion III Interface (ThermoQuest Finnigan). The GC was fitted with a GS-Carbonplot capillary column (30 m × 0.32 mm i.d., d f 1.5 μm; Agilent Technologies) and a PoraPlot capillary column (25 m × 0.25 mm i.d., d f 8 μm; Varian, Lake Forest, USA). The columns were coupled using a press fit connector. Aliquots of headspace gas from samples were transferred to an evacuated sample loop (40 ml). CH 4 was separated from interfering compounds by GC, trapped on Hayesep D and then transferred to the GC-C-IRMS system. All 13 C/ 12 C isotope ratios ( δ 13 C values) are expressed in the conventional δ notation in per mil versus VPDB, defined as: A tank of high-purity carbon dioxide (carbon dioxide 4.5, Messer Griesheim, Frankfurt, Germany) with a known δ 13 C value of −23.63‰ (VPDB) was used as the working reference gas. All δ 13 C values obtained from analysis of CH 4 were corrected using three CH 4 working standards (Isometric Instruments, Victoria, Canada) calibrated against International Atomic Energy Agency and NIST reference substances. The calibrated δ 13 C values of the three working standards in ‰ versus VPDB were −23.9±0.2, −38.3±0.2 and −54.5±0.2‰. Samples were routinely analysed three times ( n =3) and average s.d. of CH 4 δ 13 C values ranged from 0.1 to 0.3‰. Methionine isotope labelling experiments Position-specific 13 C labelling experiments were conducted with methionine that had a significant 13 C enrichment of the carbon atom of the thio-methyl group. Preparation of 13 C-enriched 13 CH 3 -MET was performed by gravimetrically mixing of 13 CH 3 -MET (Sigma-Aldrich, Taufkirchen, Germany; Isotec 99% 13 C atoms) with unlabelled MET (Sigma-Aldrich; CAS number 63-68-3, 1.07% 13 C atoms) at a ratio of 1:99. Based on the ratio of gravimetrical mixing, the amount of 13 C in the thio-methyl group was calculated to be 2±0.05%, corresponding to a δ 13 C (- S -methyl- 13 C) value of 822±50‰. The measured and corrected δ 13 C(CH 4 ) value for the headspace gas of the sample was 763±16‰, and thus reflected closely the δ 13 C(- S -methyl- 13 C) value of the isotopically labelled thio-methyl group. δ 13 C(CH 4 ) value of the background (laboratory air) was −46.1±0.3‰. Tobacco plants cultivated under sterile conditions The medium used for tobacco plants ( N. tabacum ) was as follows: 4.56 g l −1 MS salts, 20 g l −1 sucrose and 10 g l −1 (plant) agar. The pH of all media was adjusted to 5.8 using KOH. Media was placed into purpose-made glass vials that were fitted with a sampling side port sealed with a hole-type screw cap containing a PTFE/silicone septum. An apical cutting of N. tabacum grown under sterile conditions was placed in the medium through the opening at the top, the opening covered with aluminium foil and the vial placed under a light relay (150 μE m −2 s −1 ) with 14 h daylight phase. Experiments were conducted after rooting when plants had grown to ~\n8–10 cm under indoor low-light conditions with no UV contribution. Supplementation of tobacco plants with 13 C methionine Tobacco plants were grown in the vials described above. Leaf infiltration ( cf . Voinnet et al. ) [53] was carried out by infiltrating 0.3 ml of a 50 mM or 10 μM 13 C methionine (99% 13 C-MET) solution into the abaxial air spaces of the plants. For root application, the growth medium was first removed from the roots, and the plants were carefully placed inside a sterile glass beaker containing 15 ml 13 C-MET solution (30 μM) such that only the roots were in direct contact with the solution. Plants and beakers were placed inside the glass vials described above. Control samples were prepared in the same way using unlabelled MET solution. After each treatment, the vials were closed using a glass plate and an O-ring fixed with a clamp and placed under the light relay at 24±1 °C. For isotope measurements, the incubation flask was directly connected to the IRMS system. Oxygen measurements An oxygen microoptode (PreSens, Regensburg, Germany; measurement based on dynamic fluorescence quenching) was used to continuously measure the oxygen concentration (μM) in the headspace or aqueous solution of the sample. Two-point calibrations were performed; argon and lab air were used to calibrate the 0 and 100% air saturation points. Hundred percent atmospheric saturation (~\n21% O 2 in lab air) corresponds to ~\n260 μM O 2 in aqueous solution (25 °C). Before the start of the experiment both the headspace and the medium were in equilibrium at ~\n260 μM O 2 . EPR measurements Continuous-wave X-band EPR spectra (ca. 9 GHz) at ambient temperature (298 K; the solutions were measured in a capillary cell) were performed on a Bruker Biospin Elexsys E500 EPR spectrometer fitted with a super high Q cavity. The magnetic field and the microwave frequency were calibrated with a Bruker ER 041XK Teslameter and a Bruker microwave frequency counter. The spin trap DMPO was purchased from Sigma-Aldrich. The DMPO solution was purified with activated charcoal, filtered and verified for the absence of EPR signals caused by contamination. All EPR samples were measured 10 min after preparation. The simulated and experimental spectra were visualized with Bruker’s Xepr software suite [54] . The experimental spectra were simulated with the computer simulation software packages XSophe-Sophe-XeprView [54] . Mass analysis Samples were neutralized with NaOH and centrifuged for 5 min at 14,000 r.p.m. The supernatant liquid was transferred, centrifuged again at 2,000 r.p.m. for 10 min and then an aliquot removed for MS analysis. LC–TOFMS analyses were conducted using an Agilent 1100 series high-performance liquid chromatography coupled to an Agilent 6510 Q-TOF (Agilent Technologies). Chromatography was performed using a reverse phase column (Agilent Eclipse Plus C18, 5 μm, 150 × 2.1 mm) together with the corresponding guard column (5 μm, 12.5 × 2.1 mm). The mobile phase consisted of 95% methanol containing 0.1% formic acid in channel A, and 5% methanol containing 0.1% formic acid in channel B. The system was programmed to perform an analysis cycle consisting of 100% B for 1 min, followed by gradient elution from 100 to 5% B over a 14-min period, hold at 5% B for 10 min, return to initial conditions over 2 min and then hold these conditions for a further 8 min. The flow rate was 0.20 ml min −1 and the injection volume was 5 μl. The MS experiments were carried out using ESI in positive ion mode with the capillary voltage set at 4.0 kV. The desolvation gas was nitrogen set at a flow rate of 8 l min −1 and maintained at a temperature of 350 °C. How to cite this article: Althoff, F. et al. Abiotic methanogenesis from organosulphur compounds under ambient conditions. Nat. Commun. 5:4205 doi: 10.1038/ncomms5205 (2014).